Giant magnetic splitting inducing near-unity valley polarization in van der Waals heterostructures Monolayers of semiconducting transition metal dichalcogenides exhibit intriguing fundamental physics of strongly coupled spin and valley degrees of freedom for charge carriers. While the possibility of exploiting these properties for information processing stimulated concerted research activities towards the concept of valleytronics, maintaining control over spin–valley polarization proved challenging in individual monolayers. A promising alternative route explores type II band alignment in artificial van der Waals heterostructures. The resulting formation of interlayer excitons combines the advantages of long carrier lifetimes and spin–valley locking. Here, we demonstrate artificial design of a two-dimensional heterostructure enabling intervalley transitions that are not accessible in monolayer systems. The resulting giant effective g factor of −15 for interlayer excitons induces near-unity valley polarization via valley-selective energetic splitting in high magnetic fields, even after nonselective excitation. Our results highlight the potential to deterministically engineer novel valley properties in van der Waals heterostructures using crystallographic alignment. The materials combined in the studied heterostructure are monolayers of transition metal dichalcogenides (TMDCs) where MX 2 denotes M = Mo, W and X = S, Se, Te. These systems were shown to host direct optical transitions in the visible spectral range at two inequivalent valleys in momentum space, labeled K+ and K−, which are situated at the corners of the hexagonal Brillouin zone [1] , [2] , [3] . Since spin and valley index of charge carriers are coupled at the K points due to the broken inversion symmetry in the monolayer combined with strong spin–orbit coupling, it is possible to selectively address and read out the valley index optically by helicity-resolved measurements [4] , [5] , [6] , [7] . However, as the two valleys are linked by time-reversal symmetry, external fields are required to break their energy degeneracy, an issue of central importance for future valleytronic devices. Recently, the effective manipulation of the valley pseudospin energy has been demonstrated for monolayer TMDCs by magnetic [8] , [9] , [10] , [11] , [12] , [13] , [14] , [15] and electric fields [16] , [17] . However, the extremely short lifetimes of excitons [18] , [19] and the fast polarization dephasing mechanisms [20] render the implementation of individual TMDC monolayers challenging for valleytronics. At the same time, the rapid development of transfer techniques has opened up a vast parameter space of artificial van der Waals heterostructures, where different two-dimensional (2D) materials are deterministically stacked upon each other [21] . For TMDCs, the resulting type II band alignment and subsequent rapid charge transfer [22] leads to the formation of interlayer excitons (IEXs), where electrons and holes are situated in different layers [23] , [24] , [25] , [26] , [27] , [28] . For stacking angles close to 0° (AA stacking) and 60° (AB stacking), negligible momentum mismatch allows radiative recombination of charge carriers at the K points [29] , [30] , leading to pronounced light emission from IEXs below the energies of the individual monolayer transitions. Nevertheless, due to the spatial separation, the wavefunction overlap in the out-of-plane direction is reduced, facilitating the potential for long lifetimes of the interlayer excitons in 2D heterostructures [27] , further supplemented by the possibility of spin–valley injection in close analogy to the monolayer systems [28] . Here, we show that the specific alignment of atomically thin layers in a heterostructure leads to intriguing fundamental physics, exclusive for such artificial systems and allowing for highly efficient external manipulation of the spin–valley degrees of freedom. In particular, we demonstrate that the magnetic coupling of electronic transitions can be strongly enhanced in AB-stacked TMDC heterobilayers, exhibiting a giant magnetic valley splitting with an effective g factor ( g eff ) of about −15 that exceeds typical values for both TMDC monolayers and more conventional nonmagnetic semiconductor heterostructures by far. Of central consequence is the resulting field-induced valley polarization of the long-lived charge carriers, even though both valleys in the two constituent materials are initially equally populated. The degree of polarization reaching near-unity values arises entirely due to the strong degeneracy lifting under magnetic fields. It emerges from the specific arrangement of the individual layers of our heterostructure in momentum space, which is not attainable in TMDC monolayer systems, enabling momentum-allowed optical transitions between valleys of different index. This leads to a situation where the sum of conduction- and valence-band valley magnetic moments contributes to significantly enhance the valley splitting in an external magnetic field compared to a monolayer system. Characterization of the WSe 2 /MoSe 2 heterostructure The heterostructure under study (shown in Fig. 1a ) consists of a monolayer of WSe 2 transferred on top of a MoSe 2 monolayer, exfoliated onto a SiO 2 /Si substrate. During the transfer process, the well-cleaved axes of the monolayers are deterministically aligned parallel to each other, ensuring a twist angle of either nearly 0° or 60°. The relative angle of the stacking configuration is confirmed through spatially resolved second-harmonic generation (SHG) spectroscopy [31] . 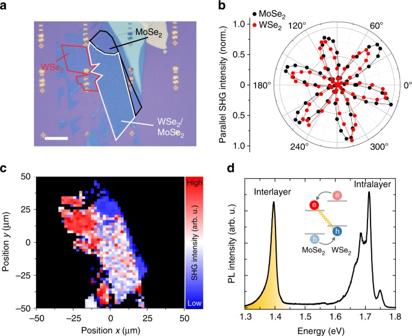Fig. 1 Interlayer excitons in a WSe2/MoSe2heterostructure with nearly 60° angle alignment.aOptical micrograph of the WSe2/MoSe2heterostructure under study. The white framed area depicts the region where the two materials overlap vertically. The scale bar is 25μm.bAngle-dependent plot of the parallel component of the SHG intensity of the individual monolayers, indicating the armchair directions of the monolayers. The relative angle between the monolayers amounts to about 54°.cSpatial scan of the sample where the total SHG intensity is recorded for each datapoint. The region of the heterostructure shows clear destructive interference of the SHG signal with respect to the individual layers.dPL spectrum taken on the heterostructure at 4 K. The emission stemming from interlayer excitons is spectrally well separated from the intralayer luminescence. The inset schematically depicts the type II band alignment of the heterostructure which leads to a spatial separation of electrons and holes Figure 1b illustrates the intensity of the parallel component of the SHG signal of the two individual monolayer materials in a polar plot. By fitting the data with a cos 2 (3 θ ) function we directly obtain a relative stacking angle θ of either 6 ± 1° or 54 ± 1° (the two possibilities stem from the phase insensitivity of the SHG intensity measurement on a single layer). To clarify the precise alignment, we perform a spatial scan of the resulting heterostructure where the total SHG intensity is recorded at each position, as shown in Fig. 1c . In the overlapping region of the two layers denoted by the white framed area in Fig. 1a , we clearly observe a pronounced destructive interference of the SHG signal with respect to the individual monolayers, consistent with a nearly 60° stacking configuration [31] . Thus, we conclude that the sample has an AB-like stacking configuration with a relative angle of 54 ± 1°. Fig. 1 Interlayer excitons in a WSe 2 /MoSe 2 heterostructure with nearly 60° angle alignment. a Optical micrograph of the WSe 2 /MoSe 2 heterostructure under study. The white framed area depicts the region where the two materials overlap vertically. The scale bar is 25μm. b Angle-dependent plot of the parallel component of the SHG intensity of the individual monolayers, indicating the armchair directions of the monolayers. The relative angle between the monolayers amounts to about 54°. c Spatial scan of the sample where the total SHG intensity is recorded for each datapoint. The region of the heterostructure shows clear destructive interference of the SHG signal with respect to the individual layers. d PL spectrum taken on the heterostructure at 4 K. The emission stemming from interlayer excitons is spectrally well separated from the intralayer luminescence. The inset schematically depicts the type II band alignment of the heterostructure which leads to a spatial separation of electrons and holes Full size image A characteristic photoluminescence (PL) spectrum of the heterostructure recorded at 4 K is shown in Fig. 1d . In line with recent reports, it consists of two separate spectral regions: [27] , [28] The intralayer transitions between 1.6 and 1.8 eV result from intralayer excitonic recombination in the constituent monolayers (WSe 2 and MoSe 2 ). At the same time, as depicted in the inset of Fig. 1d , rapid charge transfer leads to the formation of interlayer excitons at around 1.4 eV, significantly lower in energy than the intralayer transitions (Additional characterization measurements are presented in Supplementary Note 1 ). Magneto-PL measurements of the interlayer exciton We now turn to the valley-resolved measurements of the interlayer transitions in an out-of-plane magnetic field (Faraday geometry). The optical experiments are carried out by exciting the sample with linearly polarized light (laser energy 1.94 eV), initially populating both valleys in the two monolayer constituents of the heterostructure equally. The emission is subsequently analyzed in a circularly polarized basis, allowing us to directly access the resulting valley-selective splitting of the transitions and quantify the degree of polarization. 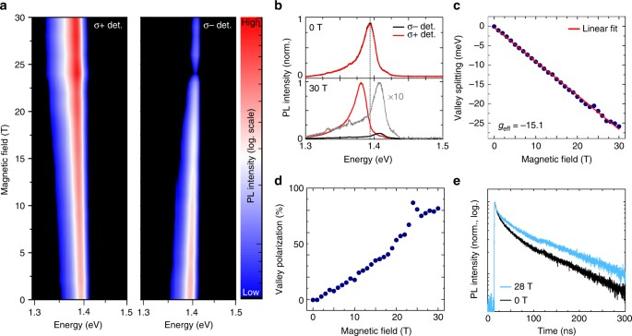Fig. 2 Magnetic field dependence of interlayer excitons.aFalse color representation of the interlayer exciton PL forσ+ andσ− polarized detection as a function of out-of-plane magnetic field up to 30 T. The excitation is performed with linearly polarized light. For better clarity the PL intensity is plotted on a logarithmic scale.bComparison of PL spectra of the interlayer exciton for 0 T and 30 T. At 0 T, both polarizations show the same energy and intensity. At 30 T, the energy degeneracy is fully lifted and the emission stems almost exclusively from theσ+ transition.cCorresponding valley-selective splitting of the interlayer exciton. The solid line corresponds to a linear fit of the data, yielding an effectivegfactor of −15.1 ± 0.1.dMagnetic-field-induced valley polarization of the interlayer exciton.eTime-resolved PL of the interlayer exciton forB= 0 T andB= 28 T Figure 2a shows the spectral evolution of the interlayer excitons for both detection polarizations in magnetic fields up to 30 T. Two main observations are immediately apparent from the data. First, the peak energy degeneracy of the interlayer transitions is lifted for fields B > 0. For rising magnetic fields, the energy of the σ + polarized component decreases monotonically while it increases for the σ − polarized component. Second, the intensity of the interlayer exciton strongly depends on the detected polarization in the magnetic field. The σ + and σ − polarized components exhibit a drastic increase and decrease in intensity, respectively, as the magnetic field is increased. These observations are further illustrated in Fig. 2b , where the two polarization configurations for B = 0 T and B = 30 T are directly compared. While at B = 0 T the two circularly polarized emission peaks are of same energy and intensity, the energy splitting between the two valley configurations amounts to about 26 meV for B = 30 T, exceeding the linewidth of the two transitions. Also, the luminescence stems almost exclusively from the σ + transition, with the σ − emission being strongly suppressed. Fig. 2 Magnetic field dependence of interlayer excitons. a False color representation of the interlayer exciton PL for σ + and σ − polarized detection as a function of out-of-plane magnetic field up to 30 T. The excitation is performed with linearly polarized light. For better clarity the PL intensity is plotted on a logarithmic scale. b Comparison of PL spectra of the interlayer exciton for 0 T and 30 T. At 0 T, both polarizations show the same energy and intensity. At 30 T, the energy degeneracy is fully lifted and the emission stems almost exclusively from the σ + transition. c Corresponding valley-selective splitting of the interlayer exciton. The solid line corresponds to a linear fit of the data, yielding an effective g factor of −15.1 ± 0.1. d Magnetic-field-induced valley polarization of the interlayer exciton. e Time-resolved PL of the interlayer exciton for B = 0 T and B = 28 T Full size image For the quantitative analysis of the data, we use Gaussian fit functions, and extract the PL peak positions of the interlayer transition for both polarizations as function of the magnetic field. The resulting valley splitting, presented in Fig. 2c , clearly follows a linear dependence. Using the definition of the splitting as Δ E IEX = E σ + − E σ − = g eff μ B B , where μ B is the Bohr magneton (≈58 μeV/T), we extract g eff = −15.1 ± 0.1 for the interlayer exciton. The corresponding degree of the valley polarization, defined as \(P = \left( {I_{\sigma ^ + } - I_{\sigma ^ - }} \right)/\left( {I_{\sigma ^ + } + I_{\sigma ^ - }} \right)\) , is presented in Fig. 2d . While it is strictly zero at B = 0, as expected, the emission is strongly polarized under the external magnetic field, exceeding values of 80% for the highest fields up to 30 T (see Supplementary Note 2 for a discussion of the enhanced valley polarization in the data around B = 24 T). We further note that such overall high degree of field-induced polarization is particularly remarkable given the fact that both valleys are initially equally populated in the experiment. Using time-resolved PL measurements (see Methods) we also track the decay dynamics of the interlayer exciton in the magnetic field. The sample is excited linearly and the total PL intensity is detected. The data are presented in Fig. 2e . The decay dynamics exhibit a complex nonexponential decay, with a 1/ e time constant of about 40 ns at 0 T followed by a longer decay (>100 ns) at later times and exceeding typical values for individual TMDC monolayers by several orders of magnitude. The lifetime further increases with rising magnetic field, with the 1/ e constant reaching 70 ns at 28 T and the longer component increasing beyond 200 ns (see Supplementary Note 3 for more detailed data). Applying an external magnetic field therefore allows us to not only to generate strongly valley-polarized carriers, but also maintain the interlayer emission on very long timescales. The determined value of about −15 for the effective g factor of the interlayer exciton is in stark contrast to experimentally determined effective g factors of excitons in individual TMDCs, found to be around −4 in most cases [9] , [10] , [11] , [12] , [14] , [15] . As we show in the following, this anomalously high effective g factor results from spin-allowed intervalley transitions in our AB-stacked heterostructure, which enables us to access novel valley physics in an external magnetic field. In monolayers, the magnitude of the magnetic coupling is often understood in terms of a simplified semiquantitative model, including three contributions, namely the spin, the atomic orbitals, and the valley magnetic moment [8] , [9] , [10] , [11] , [12] . Since the optical transitions are spin conserving between conduction and valence band, the net contribution from the spin to the energy splitting of the respective resonances is zero. On the other hand, only the valence bands carry a non-zero magnetic moment μ l from the atomic orbitals with μ l = 2 for the K+ valley and μ l = −2 for the K− valley, leading to an overall splitting between the valley-selective transitions of −4 μ B B . The third contribution, the valley magnetic moment μ k , arises from the self-rotation of the Bloch wavepackets [32] . It is defined by \( \pm \mu _k^c = m_0/m_e\) for the conduction band and \( \pm \mu _k^v = m_0/m_h\) for the valence band in the K+/K− valley, respectively. As the optically allowed transitions in a monolayer take place between valleys of the same index (intravalley), these contributions cancel out almost entirely. For intervalley transitions in a monolayer system, the contributions from the valley magnetic moments add up, leading to higher g factors [33] . These transitions cannot be optically accessed in a pristine monolayer system due to their high momentum mismatch. However, they may be responsible for the large g factors observed in defect-related emission [34] , [35] , [36] , [37] , [38] . Therefore, the total field-induced magnetic shift for a monolayer TMDC can be written as Δ E 1L = E σ + − E σ − = −(4−2( m 0 / m e − m 0 / m h )) μ B B ≈ −4 μ B B , as m h ≈ m e in many cases. The deviations from this value are attributed both to nonequivalent effective masses of electrons and holes and the complexities of the orbital contributions to the energetic shift beyond the simplified model [12] . In an AB-stacked heterostructure, however, we encounter a markedly different situation for optically bright transitions. 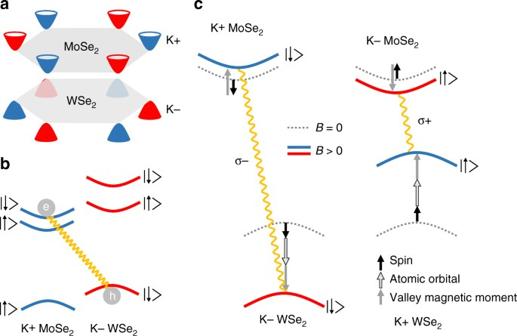Fig. 3 Giant magnetic valley splitting in an AB-stacking configuration.aMomentum space arrangement of the relevant band extrema in an AB-stacked WSe2/MoSe2heterostructure. Blue (red) depicts electronic bands from the K+ (K−) valleys.bType II band alignment of MoSe2and WSe2for the AB-stacking configuration, indicating spin-allowed optically bright interlayer transitions. Arrows indicate spin-up and spin-down states.cEvolution of the transitions such as indicated inbwith positive applied magnetic field. Dashed lines indicate the situation forB= 0. The arrows depict the possible contributions to the valley-selective splitting (black for spin, black framed for atomic orbital and gray for valley magnetic moment) Figure 3a schematically depicts the configuration of the Brillouin zones for interlayer excitons in an AB-stacked WSe 2 /MoSe 2 heterostructure. Here, the optical transitions take place between the K− valley of WSe 2 and the K+ valley of MoSe 2 (and by symmetry, also from K+ in WSe 2 to K− in MoSe 2 ). Hence, in contrast to monolayer systems, the optical transitions are not valley conserving for AB-stacked heterobilayers. This is further illustrated in Fig. 3b which shows one of the two interlayer transitions. After the optical excitation and following fast charge transfer, electrons in the upper conduction band of MoSe 2 reside in the K+ valley whereas the holes in WSe 2 are located in the K− valley (here, we use the convention where the vacant electron states and the corresponding holes in the valence band are defined to have the same momenta). This configuration, in analogy to tungsten-based monolayer TMDCs, leads to the spin-allowed and optically bright transitions involving the upper conduction band of MoSe 2 while a transition from the lower conduction band is not spin conserving and thus optically dark. The anomalous situation in momentum space directly impacts the valley splitting of the interlayer exciton in an external magnetic field, which is schematically depicted in Fig. 3c . Fig. 3 Giant magnetic valley splitting in an AB-stacking configuration. a Momentum space arrangement of the relevant band extrema in an AB-stacked WSe 2 /MoSe 2 heterostructure. Blue (red) depicts electronic bands from the K+ (K−) valleys. b Type II band alignment of MoSe 2 and WSe 2 for the AB-stacking configuration, indicating spin-allowed optically bright interlayer transitions. Arrows indicate spin-up and spin-down states. c Evolution of the transitions such as indicated in b with positive applied magnetic field. Dashed lines indicate the situation for B = 0. The arrows depict the possible contributions to the valley-selective splitting (black for spin, black framed for atomic orbital and gray for valley magnetic moment) Full size image In analogy to the monolayer system, the contribution to the valley splitting from spin cancels out and the magnetic moment from the atomic orbitals μ l in the valence bands results in an expected energetic splitting of −4 μ B B . The contributions from the valley magnetic moments μ k , however, now have the opposite sign for the conduction and valence bands and thus add up instead of canceling out as it is the case for individual monolayers. This signifies the main magnetic property of the interlayer transitions in AB-stacked heterostructures with the energetic shifts of the valley magnetic moments evolving antiparallel in the conduction and valence bands in a magnetic field. For the σ − transition in Fig. 3c this leads to a drastic increase of the transition energy when a magnetic field is applied. For the same reasons, a strong decrease occurs for the σ + transition, since the two valley configurations are linked by time-reversal symmetry. The total valley-selective splitting of the interlayer transition Δ E IEX induced by the magnetic field then amounts to Δ E IEX = E σ + − E σ − = −(4 + 2( m 0 / m e + m 0 / m h )) μ B B . Using calculated values [39] for the effective masses of electrons ( m e = 0.57 m 0 ) in the upper conduction band of MoSe 2 and holes ( m h = 0.36 m 0 ) in the valence band of WSe 2 we obtain g eff = −13.1 for the interlayer transition, in close agreement with the experimentally determined value of g eff = −15.1 ± 0.1. The presence of large band offsets in TMDC heterostructures combined with the angle alignment of the nonequivalent valleys thus yields interlayer transitions with an unusually large total effective g factor, which is a powerful lever to exploit the valley degree of freedom. Even higher effective g factors can be expected when suitable van der Waals materials with lower effective masses are combined. Thus, even for nonselective injection with respect to spin–valley degrees of freedom, strong spin–valley polarization in an applied magnetic field is expected already at thermal equilibrium steady-state conditions, as demonstrated in our experiment. This finding is of particular importance when-above bandgap optical excitation or electrical injection are considered, both being most common scenarios in devices. Additionally, we envision the use of local (stray or exchange) magnetic fields generated by microstructured ferromagnets to define valley-selective potential landscapes for interlayer excitons. These local, valley-selective potentials may be used to filter or trap excitons with a specific valley polarization, and the large energy splitting resulting from the effective g factor will enable operation of such devices well above liquid-helium temperatures. Finally, the demonstrated stability of the spin–valley polarization through the complete lifting of valley degeneracy in artificial heterostructures provides a highly promising route towards the implementation of the spin–valley degree of freedom for future applications in the fields of quantum computation and nanophotonics. Sample fabrication The WSe 2 /MoSe 2 heterostructure was fabricated by means of an all-dry transfer procedure [40] on a Si/SiO 2 substrate. The constituent monolayer samples were obtained by mechanical exfoliation of bulk crystals (HQGraphene). After the transfer process, the sample was annealed for 5 h at 150 °C in high vacuum. Second-harmonic generation spectroscopy SHG measurements were carried out at room temperature with a Ti:sapphire laser (pulse length 100 fs, central wavelength 810 nm) focused on the sample via a 40 × microscope objective. The signal was coupled into a grating spectrometer and detected with a CCD camera. For polarization-dependent measurements, the laser light was linearly polarized and the reflected light was analyzed by the same polarizer, thereby selecting the parallel signal component of the SHG. The sample was rotated by a mechanical stage in order to obtain angle resolution. For mapping of the total SHG intensity, the sample was excited using circularly polarized light without any polarization analysis in the detection. The sample was scanned under the microscope using a motorized x–y stage and the total SHG intensity was recorded for each sample position. Magneto-PL spectroscopy The sample was placed on a x–y–z piezoelectric stage and cooled down to 4.2 K in a cryostat filled with liquid helium. Magnetic fields up to 30 T were applied by means of a resistive magnet in Faraday configuration. For static PL measurements, laser light at an energy of 1.94 eV was focused onto the sample with a microscope objective resulting in a spot size of ~4μm. The polarization of the PL was analyzed with a quarter-wave plate and a linear polarizer. Using a nonpolarizing beam splitter, the backscattered PL was guided to the spectrometer and detected with a liquid nitrogen-cooled CCD. Time-resolved PL measurements were carried out with a pulsed diode laser (laser energy 1.80 eV, repetition rate 2.5 Mhz) which was synchronized to an avalanche photodiode. The PL from the interlayer exciton was spectrally selected with a longpass filter. Data availability The data that support the findings of this study are available from the corresponding authors upon request.